PGD2deficiency exacerbates food antigen-induced mast cell hyperplasia Prostaglandin D 2 (PGD 2 ) is a major prostanoid secreted mainly by mast cells. Although PGD 2 has been identified as a modulator of allergic inflammation, its precise role remains unclear. Here we investigate the role of PGD 2 in food allergy. Oral administration of ovalbumin induces allergic responses in sensitized wild-type (WT) mice. Systemic gene deficiency of haematopoietic PGD synthase ( H-PGDS −/− ) exacerbates all of the manifestations accompanying severe mast cell hyperplasia in the intestine. Morphological studies show that c-kit/FcɛRI-positive WT mast cells strongly express H-PGDS. Transplantation of H-PGDS −/− mast cells also aggravates ovalbumin-induced mast cell hyperplasia and allergic symptoms in mast cell null mice. H-PGDS deficiency accelerates the production of SDF-1α and the activity of MMP-9 in the antigen-stimulated intestine. SDF-1α receptor blockade or MMP-9 inhibition relieves the exacerbated mast cell hyperplasia and manifestations observed in H-PGDS −/− . Thus, PGD 2 deficiency results in food antigen-induced mast cell hyperplasia. Food allergy is defined as an abnormal immune response to food proteins. The number of patients with food allergies has doubled within the last several decades. Currently, 2–10% of the human population suffers from hypersensitivity to certain food proteins [1] . Symptoms affecting the skin, lung and gastrointestinal (GI) tract include eczema, laboured breathing and diarrhoea. In serious cases, hypersensitivity to food antigens may lead to systemic anaphylaxis reactions, thus threatening the life of the patient. Since few effective treatments are available for these reactions, the remaining option for patients is to avoid the causative antigens (that is, specific foods). Therefore, the development of new clinical applications for food allergies is urgently needed. Mast cells are major players in allergic diseases. Following the onset of inflammation, several chemoattractants are produced that stimulate the release of mast cell progenitors (MCps) from bone marrow (BM) into the circulation [2] . Circulating MCps migrate and mature peripherally in connective or mucosal tissues. Stem cell factor (SCF) plays a central role in chemoattraction and the proliferation and maturation of MCps [3] . Stromal-derived factor (SDF)-1α and tumour necrosis factor (TNF)-1α are also known to induce migration of MCps into peripheral tissues [4] . In the sensitization phase of allergy, the uptake of a food antigen activates T- or B-lymphocytes to produce immunoglobulin E (IgE), which binds to mast cells through its high affinity receptor FcɛRI. Upon re-uptake of antigens, IgEs are crosslinked, which in turn degranulates the mast cells to release a large number of inflammatory mediators, including histamine, platelet-activator factor (PAF), cysteinyl leukotrienes (cys-LTs) and prostaglandin D 2 (PGD 2 ). The secreted histamine rapidly and strongly increases capillary permeability, whereas PAF mainly induces platelet aggregation and degranulation [5] , [6] . Mast cells strongly express haematopoietic PGD synthase (H-PGDS) and produce a large amount of the arachidonic acid metabolite PGD 2 (ref. 7 ). PGD 2 exerts its biological actions though two distinct receptors, D prostanoid (DP) and the chemoattractant receptor-homologous molecule expressed on Th2 cells (CRTH2). The dehydration product of PGD 2 , 15-deoxy-delta PGJ 2 (15d-PGJ 2 ), also has bioactivity via peroxisome proliferator-activated receptors [8] . Although PGD 2 has emerged as a mast cell-derived allergic mediator, there is uncertainty regarding its contribution to allergic inflammation. Several studies have reported a pro-inflammatory role associated with PGD 2 signalling. Inhalation of PGD 2 induced nasal blockage via the DP receptor in atopic rhinitis patients [9] . In addition, PGD 2 enhanced airway inflammation by accumulation of inflammatory cells via the DP receptor on epithelial cells [10] , [11] . Conversely, other studies have suggested anti-inflammatory roles for PGD 2 . In mouse asthma model, DP agonism reduced eosinophilia and airway hyperresponsiveness [12] , whereas CRTH2 agonism restricted the recruitment of eosinophils by limiting the production of interleukin (IL)-5 (ref. 13 ). Thus, the role of PGD 2 signalling in allergic response remains poorly understood. In this study, we investigated the role of PGD 2 in food allergy using genetically modified mice. We found that lack of PGD 2 results in food antigen-induced mast cell hyperplasia. H-PGDS deficiency exacerbates food allergy Naive H-PGDS −/− mice with a C57BL/6-background did not present any congenital GI tract abnormalities, such as changes in morphology ( Supplementary Fig. 1a,b ), epithelial permeability ( Supplementary Fig. 1c ), mRNA expression of inflammatory cytokines ( Supplementary Fig. 1d ) or tissue serotonin content, which causes oral antigen-induced diarrhoea [14] ( Supplementary Fig. 1e ). In addition, both lines of mice showed comparative hypothermia in IgE/mast cell-mediated passive systemic anaphylaxis ( Supplementary Fig. 1f ). Diarrhoea is a representative symptom in murine models of food allergy [15] . We assessed the stool consistency ( Fig. 1a ) and scored other systemic responses including scratching, immobility and swelling (bristled fur, oedema around the nose and eyes or laboured breathing; Fig. 1b ). In wild-type (WT) mice, both scores increased after the seventh or eighth oral challenge of 50 mg ovalbumin (OVA), whereas more severe symptoms with earlier onset developed in H-PGDS −/− mice. We next investigated whether H-PGDS deficiency affected serum IgE levels. Although OVA challenges significantly increased serum OVA-specific IgE levels in both WT and H-PGDS −/− mice, there was no significant difference between the lines after ten times OVA challenges ( Fig. 1c ). 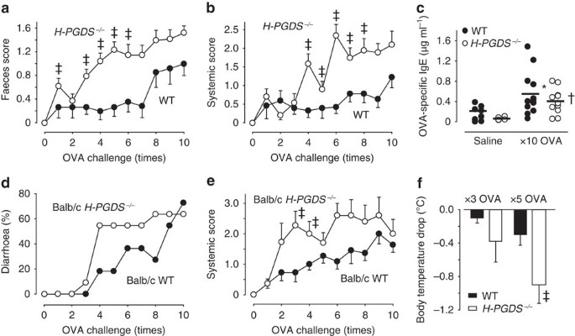Figure 1: H-PGDS deficiency exacerbates OVA-induced allergic reactions. Faeces score (a) and systemic score (b) were monitored in C57BL/6-background mice (n=8–12). (c) Serum OVA-specific IgE levels in mice following the tenth challenge with either saline or OVA (n=8–12). The horizontal lines indicate the means. Diarrhoea occurrence (d), systemic score (e) and hypothermia (f) were monitored in Balb/c-background mice (n=11). Diarrhoea occurrence is represented as the percentage over the number of OVA challenges.*, †,P<0.05 compared with saline-challenged WT, saline-challengedH-PGDS−/−or OVA-challenged WT, respectively. Data are presented as mean±s.e.m. of 2–3 independent experiments. Mann–WhitneyU-test was performed for comparisons ina,bande, and Tukey’s test for comparison incandf. Figure 1: H-PGDS deficiency exacerbates OVA-induced allergic reactions. Faeces score ( a ) and systemic score ( b ) were monitored in C57BL/6-background mice ( n =8–12). ( c ) Serum OVA-specific IgE levels in mice following the tenth challenge with either saline or OVA ( n =8–12). The horizontal lines indicate the means. Diarrhoea occurrence ( d ), systemic score ( e ) and hypothermia ( f ) were monitored in Balb/c-background mice ( n =11). Diarrhoea occurrence is represented as the percentage over the number of OVA challenges. *, †, P <0.05 compared with saline-challenged WT, saline-challenged H-PGDS −/− or OVA-challenged WT, respectively. Data are presented as mean±s.e.m. of 2–3 independent experiments. Mann–Whitney U -test was performed for comparisons in a , b and e , and Tukey’s test for comparison in c and f . Full size image Allergic responses are known to vary among mouse strains [15] . Balb/c WT mice exhibited diarrhoea even in response to 1 mg OVA ( Supplementary Fig. 2a ). At this lower dosage of OVA, Balb/c H-PGDS −/− showed earlier and more severe manifestations including diarrhoea ( Fig. 1d ), systemic reactions ( Fig. 1e ) and hypothermia ( Fig. 1f ) than that observed in WT mice. A higher dosage of OVA (10 mg) caused comparable diarrhoea occurrence in both lines of Balb/c mice ( Supplementary Fig. 2b ). Thus, H-PGDS deficiency exacerbated food allergy regardless of the mouse strain. C57BL/6 mouse lines were utilized for the subsequent experiments. H-PGDS deficiency exacerbates mast cell infiltration Mast cells are located at the sites exposed to external environment such as GI tract and skin. We counted the infiltrated mast cells visualized by chloroacetate esterase (CAE) staining in small and large intestine, and also in lung and ear. The number of mast cells in those tissue was no difference between both lines of mice before OVA stimulation ( Supplementary Fig. 3a ). OVA challenge stimulated mast cell infiltration into the intestinal tract as well as in the other sites in WT ( Fig. 2a ). H-PGDS deficiency was observed to accelerate mast cell infiltrations, resulting in mast cell hyperplasia in almost all of the tissues ( Fig. 2a ). In both humans and mice, mast cells accumulate around the GI tract during the progression of food allergy, which aggravates allergic manifestations [16] , [17] . Consistently, mast cell hyperplasia was especially remarkable in the colon, but was not significant in the jejunum, which was also observed in Balb/c mice ( Fig. 2a and Supplementary Fig. 3b ). In the inflamed ileums and colons, most mast cells were observed in the mucosa, particularly in the intraepithelial region and the lamina propria (middle panel, Fig. 2b ). The same observations were obtained in flow cytometric analysis ( Supplementary Fig. 3c ). Degranulating mast cells were observed with approximately the same frequency in both lines (small panel, arrowheads, Fig. 2b ), and electron micrograph analysis revealed no differences in granular cytoplasmic appearance ( Fig. 2c ). Serum mouse mast cell protease-1 (mMCPT-1), a unique mediator released from the intestinal mucosal mast cell, was also significantly upregulated in OVA-challenged H-PGDS −/− mice (× 10 OVA; Fig. 2d ). In contrast, no differences between the two lines were observed in the mRNA ( Supplementary Fig. 4a,c ) or protein ( Supplementary Fig. 4b,d ) expression of Th2 cytokines such as IL-4 and IL-13. 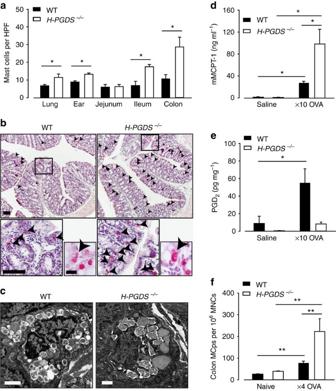Figure 2: H-PGDS deficiency accelerates the infiltration of mast cells and MCps. (a) Mean number of mast cells per high power field (HPF) in each tissue following the tenth OVA challenge (n=4–5). (b) Representative pictures of CAE-stained colon sections (× 200 and × 400 magnification; scale bars, 100 μm). Arrowheads indicate infiltrating mast cells. The small panel shows the degranulating mast cells (scale bar, 20 μm). (c) Representative pictures of transmission electron microscopy (scale bars, 2 μm) following the tenth OVA challenge for WT andH-PGDS−/−mice. Serum mMCPT-1 (d) and PGD2in the colons (e) of mice following the tenth saline or OVA challenge (n=4–5). (f) Mean number of MCps per 106MNCs in the colon of naive and fourth OVA-challenged mice (n=4–5). Data are presented as mean±s.e.m. of 2–3 independent experiments. *P<0.05, **P<0.01. Tukey’s test was performed for comparison. Figure 2: H-PGDS deficiency accelerates the infiltration of mast cells and MCps. ( a ) Mean number of mast cells per high power field (HPF) in each tissue following the tenth OVA challenge ( n =4–5). ( b ) Representative pictures of CAE-stained colon sections (× 200 and × 400 magnification; scale bars, 100 μm). Arrowheads indicate infiltrating mast cells. The small panel shows the degranulating mast cells (scale bar, 20 μm). ( c ) Representative pictures of transmission electron microscopy (scale bars, 2 μm) following the tenth OVA challenge for WT and H-PGDS −/− mice. Serum mMCPT-1 ( d ) and PGD 2 in the colons ( e ) of mice following the tenth saline or OVA challenge ( n =4–5). ( f ) Mean number of MCps per 10 6 MNCs in the colon of naive and fourth OVA-challenged mice ( n =4–5). Data are presented as mean±s.e.m. of 2–3 independent experiments. * P <0.05, ** P <0.01. Tukey’s test was performed for comparison. Full size image OVA administration resulted in increased PGD 2 content in the colons of WT mice (× 10 OVA; Fig. 2e ), which was not observed in H-PGDS −/− mice, suggesting that H-PGDS dominantly produces PGD 2 in this model. H-PGDS deficiency exacerbates MCp infiltration Circulating MCps infiltrate into peripheral tissues and mature into functionally active mast cells. We counted the tissue-infiltrated MCps that possessed the ability to differentiate into mature mast cells after cultivation with IL-3 ( Fig. 2f ). Without stimulation, a low and equivalent number of MCps was found in the colon tissues of WT and H-PGDS −/− mice (naive). OVA challenge increased the appearance of MCps in WT mice (× 4 OVA). H-PGDS deficiency further increased the number of MCps, suggesting that H-PGDS deficiency generates a favourable environment for MCps to infiltrate into the inflamed colon and aggravate mast cell hyperplasia. Infiltrated mast cells express H-PGDS Immunostaining was performed to determine which cells express H-PGDS in the allergic colons of WT mice. As expected, c-kit- and FcɛRI-positive mast cells strongly expressed H-PGDS ( Fig. 3a,b ), and ∼ 91% of c-kit-positive cells stained with H-PGDS (c-kit + ; 6.6±1.3, c-kit + H-PGDS + ; 6.0±1.3/high power field, × 400 magnification; Fig. 3c ), whereas CD11b-, CD4- and CD8-positive cells did not ( Fig. 3d–f , respectively). Consistent with observations from CAE staining, the number of c-kit-positive mast cells in the H-PGDS −/− mice was greater than that in WT mice. These results imply that mast cell-derived PGD 2 somehow modulated infiltration of the mast cells into the inflamed colon. 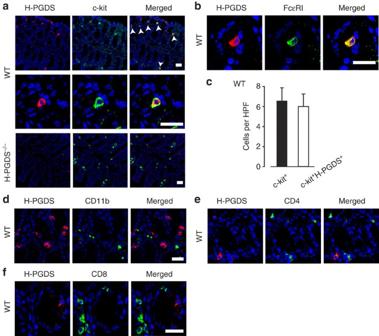Figure 3: Mast cells express H-PGDS. Representative pictures (× 200 and × 400 magnification; scale bars, 20 μm) of colon sections stained for H-PGDS and c-kit (a), FcɛRI (b), CD11b (d), CD4 (e) and CD8 (f). H-PGDS deficiency increases c-kit-positive mast cells in the colon (a, lower panels). (c) Mean number of c-kit-positive and c-kit-H-PGDS-positive cells in WT colon (n=5 each). Data are presented as mean±s.e.m. HPF, high power field. Figure 3: Mast cells express H-PGDS. Representative pictures (× 200 and × 400 magnification; scale bars, 20 μm) of colon sections stained for H-PGDS and c-kit ( a ), FcɛRI ( b ), CD11b ( d ), CD4 ( e ) and CD8 ( f ). H-PGDS deficiency increases c-kit-positive mast cells in the colon ( a , lower panels). ( c ) Mean number of c-kit-positive and c-kit-H-PGDS-positive cells in WT colon ( n =5 each). Data are presented as mean±s.e.m. HPF, high power field. Full size image H-PGDS-deficient mast cells exacerbate food allergy Kit W-sh/W-sh mice lack mature mast cells because of an inversion mutation in the Kit gene promoter. Kit W-sh/W-sh mice did not exhibit significant allergic responses, although some mice were observed to scratch their ears following the tenth OVA challenge ( Supplementary Fig. 5 ). This observation is in agreement with results of a previous study reporting a low number of mast cells residing in the ear skin of Kit W-sh/W-sh mice [18] . In this series of experiments, we evaluated the allergic responses excluding the scratch score ( Fig. 4c ). 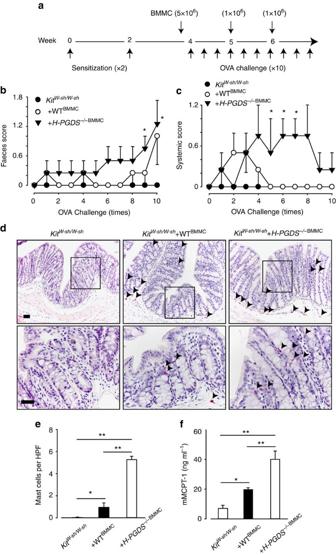Figure 4: Mast cell-specific deficiency exacerbates allergic reaction and mast cell infiltration. (a) Experimental outline. After twice sensitizations,KitW-sh/W-shmice were reconstituted with BMMC by multiple injections (three times in total). Faeces score (b) and systemic score without scratch (c) were monitored inKitW-sh/W-shmice transplanted with BMMCs by multiple injection (n=4–7). Representative pictures of CAE-stained colon sections (n=4–7; × 200 and × 400 magnification; scale bars, 50 μm) (d), mean number of mast cells per high power field (HPF) in the colon of mice (n=4–5) (e) and serum mMCPT-1 levels (n=4–5) (f) following the tenth OVA challenge. Data are presented as mean±s.e.m. *P<0.05, **P<0.01. Mann–WhitneyU-test was performed for comparisons inb,c, and Tukey’s test for comparison ine,f. Figure 4: Mast cell-specific deficiency exacerbates allergic reaction and mast cell infiltration. ( a ) Experimental outline. After twice sensitizations, Kit W-sh/W-sh mice were reconstituted with BMMC by multiple injections (three times in total). Faeces score ( b ) and systemic score without scratch ( c ) were monitored in Kit W-sh/W-sh mice transplanted with BMMCs by multiple injection ( n =4–7). Representative pictures of CAE-stained colon sections ( n =4–7; × 200 and × 400 magnification; scale bars, 50 μm) ( d ), mean number of mast cells per high power field (HPF) in the colon of mice ( n =4–5) ( e ) and serum mMCPT-1 levels ( n =4–5) ( f ) following the tenth OVA challenge. Data are presented as mean±s.e.m. * P <0.05, ** P <0.01. Mann–Whitney U -test was performed for comparisons in b , c , and Tukey’s test for comparison in e , f . Full size image In the preliminary experiments, we delivered WT or H-PGDS −/− BM-derived mast cells (BMMCs) to Kit W-sh/W-sh mice by single injection 6 weeks before OVA sensitization as previously described protocol [18] ( Supplementary Fig. 6a ). This mouse model responded to the OVA challenges but did not exhibit disease exacerbation ( Supplementary Fig. 6b,c ). Engrafted mast cells were localized in the submucosa or muscle but not in the intraepithelium and lamina propria ( Supplementary Fig. 6d ). Its number did not increase along with the challenge times observed in general WT and H-PGDS −/− mice ( Supplementary Fig. 6e ). Thus, in the current study, we performed multiple BMMC injections (three times in total) before and after the OVA stimulation every other week ( Fig. 4a ). Multiple adoptive transfer of WT BMMCs ( Kit W-sh/W-sh +WT BMMC ) caused allergic responses (+WT BMMC ; Fig. 4b,c ). Transplantation of H-PGDS −/− BMMCs ( Kit W-sh/W-sh + H-PGDS −/−BMMC ) also resulted in allergic reactions, producing higher scores than Kit W-sh/W-sh +WT BMMC throughout the experimental period (+ H-PGDS −/−BMMC ; Fig. 4b,c ). Engrafted mast cells resided in the intraepithelium or lamina propria (lower panel, arrowhead, Fig. 4d ). Notably, grafting of H-PGDS −/− BMMCs into Kit W-sh/W-sh mice colons was enhanced in comparison with that of WT BMMCs ( Fig. 4e ), which was accompanied by changes in the levels of serum mMCPT-1 ( Fig. 4f ). These observations supported the idea that PGD 2 secreted from newly infiltrated mast cells in response to antigen stimulation attenuated mast cell hyperplasia and the consequent allergic reactions. H-PGDS-derived PGD 2 inhibits mast cell chemoattractants SCF and TNF-α, LTB 4 (synthetized by 5-lipoxygenase and leukotriene A 4 hydrolase), CCL-2, SDF-1α, IL-9 and IL-3 have been identified as chemoattractants or growth cofactors for MCps [2] , [19] . In allergic colon tissues, there were no differences in the mRNA expression ( Supplementary Fig. 7a ) or protein content ( Fig. 5a ) of many of these factors, whereas SDF-1α content was significantly increased in H-PGDS −/− ( Fig. 5b ). In addition, mRNA expression ( Supplementary Fig. 7a ) and the activity ( Fig. 5c ) of matrix metalloproteinase-9 (MMP-9), which cleaves and releases SCF and TNF-α from the cell membrane [20] , [21] , were observed to increase in H-PGDS −/− mice. 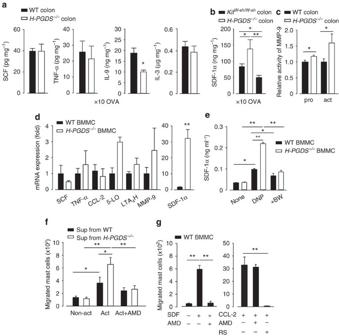Figure 5: H-PGDS deficiency accelerates SDF-1α production in mast cells. (a) The protein contents of SCF, TNF-α, IL-9 and IL-3 in the tenth OVA-challenged colon (n=4–5). Student’st-test was performed for comparison. (b) SDF-1α content in the colon of WT,H-PGDS−/−andKitW-sh/W-shfollowing the tenth OVA challenge (n=4 each).KitW-sh/W-shshowed significantly lower levels than WT orH-PGDS−/−. (c) Densitometric analysis of gelatin zymograms from tenth OVA-challenged colon for proMMP-9 (pro; 105 kDa) and activated (act) MMP-9 (88 and 95 kDa;n=4 each). (d) mRNA expression of several chemoattractants in BMMCs activated by DNP-HSA (10 ng ml−1) (n=4). The data are presented as the ratio to WT. (e) SDF-1α secretion into the culture medium of activated BMMCs (n=4–5). In some experiments, BW245C (30 nM) was pretreated 10 min before activation (n=4). Chemotaxis of WT BMMCs in response to the culture medium (supernatant: Sup) (f), SDF-1α or CCL-2 (g) of activated mast cells. The diluted supernatant (1:50), SDF-1α (100 ng ml−1) or CCL-2 (10 ng ml−1) were added to the lower chamber. After 5 h, the migrating cells collected from the lower chamber were counted using flow cytometry (n=4–8). In some experiments, AMD3100 (10 μM) or CCR2 antagonist, RS504393 (10 μM) was added to both upper and lower chambers (n=4–5). Data are presented as mean±s.e.m. *P<0.05,**P<0.01. Tukey’s test was performed for comparison inb–fand Dunnett’s test ing. Figure 5: H-PGDS deficiency accelerates SDF-1α production in mast cells. ( a ) The protein contents of SCF, TNF-α, IL-9 and IL-3 in the tenth OVA-challenged colon ( n =4–5). Student’s t -test was performed for comparison. ( b ) SDF-1α content in the colon of WT, H-PGDS −/− and Kit W-sh/W-sh following the tenth OVA challenge ( n =4 each). Kit W-sh/W-sh showed significantly lower levels than WT or H-PGDS −/− . ( c ) Densitometric analysis of gelatin zymograms from tenth OVA-challenged colon for proMMP-9 (pro; 105 kDa) and activated (act) MMP-9 (88 and 95 kDa; n =4 each). ( d ) mRNA expression of several chemoattractants in BMMCs activated by DNP-HSA (10 ng ml −1 ) ( n =4). The data are presented as the ratio to WT. ( e ) SDF-1α secretion into the culture medium of activated BMMCs ( n =4–5). In some experiments, BW245C (30 nM) was pretreated 10 min before activation ( n =4). Chemotaxis of WT BMMCs in response to the culture medium (supernatant: Sup) ( f ), SDF-1α or CCL-2 ( g ) of activated mast cells. The diluted supernatant (1:50), SDF-1α (100 ng ml −1 ) or CCL-2 (10 ng ml −1 ) were added to the lower chamber. After 5 h, the migrating cells collected from the lower chamber were counted using flow cytometry ( n =4–8). In some experiments, AMD3100 (10 μM) or CCR2 antagonist, RS504393 (10 μM) was added to both upper and lower chambers ( n =4–5). Data are presented as mean±s.e.m. * P <0.05, ** P <0.01. Tukey’s test was performed for comparison in b – f and Dunnett’s test in g . Full size image We next investigated the characteristic changes in mast cells resulting from H-PGDS deficiency. H-PGDS −/− BMMCs presented the same proliferation ( Supplementary Fig. 8a ), maturation (FcɛRI expression; Supplementary Fig. 8b ) and function (degranulation rate and cys-LTs production; Supplementary Fig. 8c,d ) as WT BMMCs. In contrast, H-PGDS deficiency increased the mRNA expression of SDF-1α in antigenically stimulated BMMCs by >20-fold compared with WT ( Fig. 5d ), whereas a less significant increase was observed for MMP-9 expression in BMMCs. H-PGDS deficiency also increased antigen-induced SDF-1α protein production in BMMCs ( Fig. 5e ). Pretreatment with a DP agonist (BW245C, 30 nM) inhibited the enhancement of SDF-1α production in both lines of BMMCs, whereas pretreatment with a degradation product of PGD 2 (15d-PGJ 2 , 30 nM) did not inhibit the enhancement of SDF-1α production (WT, 98.3±11.8; H-PGDS −/− , 196.7±28.4 pg ml −1 ). Therefore, mast cell-derived PGD 2 appears to suppress the production of SDF-1α via DP-mediated signalling. Mast cell-derived PGD 2 suppresses chemoattractant production We next focused on the contribution of hypersecreted SDF-1α to mast cell recruitment under conditions of H-PGDS deficiency. In the in vitro chemotaxis assay, the culture medium (supernatant) of antigenically activated WT BMMCs induced a chemotactic response ( Fig. 5f ). The supernatant of activated H-PGDS −/− BMMCs exhibited a stronger chemotactic response than that of WT BMMCs. SDF-1α is known to stimulate mast cell migration by activating CXC chemokine receptor type 4 (CXCR4; ref. 22 ). Treatment with a specific CXCR4 antagonist [23] (AMD3100, 10 μM) attenuated the chemotactic ability of the supernatant of activated H-PGDS −/− BMMCs. AMD (10 μM) specifically inhibited WT BMMC migration induced by SDF-1α (100 ng ml −1 ) alone but not that induced by another chemokine, CCL-2 (10 ng ml −1 ; Fig. 5g ). Finally, we examined the inhibition of CXCR4 or MMP-9 in food antigen-induced mast cell hyperplasia in vivo . AMD (300 μg per mouse) completely suppressed increases in faeces scores (+AMD; Fig. 6a ) and inhibited the infiltration of mast cells ( Fig. 6b ) and MCp ( Fig. 6c ) in both WT and H-PGDS −/− colons. AMD also suppressed the systemic scores in H-PGDS −/− but had less pronounced effects on the systemic scores of WT mice ( Supplementary Fig. 9 ). Adoptive transfer of CXCR4 −/− BMMCs into Kit W-sh/W-sh mice resulted in a lower faeces scores than that in WT mice at the tenth OVA challenge (WT BMMC ; 1.0±0.6, CXCR4 −/−BMMC ; 0.2±0.2, n =4–5) and resulted in impaired engraftment of mast cells in the colon (WT BMMC ; 1.5±0.3, CXCR4 −/−BMMC ; 0.6±0.2, P <0.05 by Student’s t -test). 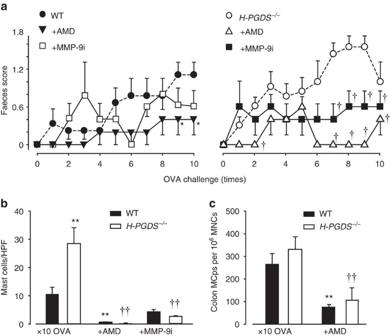Figure 6: CXCR4 antagonism or MMP-9 inhibition attenuates allergic responses and mast cell hyperplasia. (a) AMD3100 (300 μg per mouse) or MMP-9 inhibitor (50 μg per mouse) was administered to mice intraperitoneally before each OVA challenge. Faeces scores were monitored (n=5–10). (b) Mean number of mast cells per high power field (HPF) in the colon of tenth OVA-challenged mice (n=4–5). (c) Mean number of MCps per 106MNCs in the colon of tenth OVA-challenged mice (n=4–5). Data are presented as mean±s.e.m.*, †P<0.05,**, ††P<0.01 compared with OVA-challenged WT or OVA-challengedH-PGDS−/−, respectively. Mann–WhitneyU-test was performed for comparisons inaand Tukey’s test for comparison inb,c. Figure 6: CXCR4 antagonism or MMP-9 inhibition attenuates allergic responses and mast cell hyperplasia. ( a ) AMD3100 (300 μg per mouse) or MMP-9 inhibitor (50 μg per mouse) was administered to mice intraperitoneally before each OVA challenge. Faeces scores were monitored ( n =5–10). ( b ) Mean number of mast cells per high power field (HPF) in the colon of tenth OVA-challenged mice ( n =4–5). ( c ) Mean number of MCps per 10 6 MNCs in the colon of tenth OVA-challenged mice ( n =4–5). Data are presented as mean±s.e.m. *, † P <0.05, **, †† P <0.01 compared with OVA-challenged WT or OVA-challenged H-PGDS −/− , respectively. Mann–Whitney U -test was performed for comparisons in a and Tukey’s test for comparison in b , c . Full size image MMP-9 inhibition (+MMP-9i, 50 μg per mouse) suppressed the increase of the faeces scores ( Fig. 6a ) and inhibited mast cell hyperplasia ( Fig. 6b ) in H-PGDS −/− mice but not in WT mice. The serum mMCPT-1 level was also significantly decreased in H-PGDS −/− mice (vehicle; 9.1±1.6, +MMP-9i; 1.3±3.9 μg ml −1 , P <0.01 by Student’s t -test). The role of PGD 2 in allergic inflammation is controversial. Several studies have reported that PGD 2 exerts a pro-inflammatory function in allergic diseases. For example, PGD 2 was shown to reinforce airway inflammation via the DP receptor in a murine asthma model [11] , whereas a selective CRTH2 agonist was shown to exacerbate allergic asthma and atopic dermatitis [12] . In contrast to these reports, the administration of a DP agonist reduced T-cell activation and alleviated symptoms of atopic dermatitis [24] , and CRTH2 agonism restricted eosinophil infiltration in allergic airway inflammation [13] . These observations were obtained by exogenous administration of PGD 2 -associated agents both in vitro and in vivo . In the present study, we clearly demonstrate that endogenous PGD 2 signalling plays an anti-inflammatory role in allergic inflammation in genetically modified mice. The mast cell is a key effector in allergic diseases. Activated mast cells secrete a wide spectrum of preformed and de novo synthesized mediators such as histamine, PAF and LTs, resulting in the development of allergic responses [25] . Therefore, the mast cell has emerged as a therapeutic target for allergic diseases. Assem and Mongar [26] originally found that sodium cromoglycate inhibits mast cell degranulation by stabilizing the cell membrane. Sodium cromoglycate has now been established as a therapeutic agent against various types of allergic diseases such as food allergy and asthma [27] , [28] . In the present study, we identified PGD 2 as an anti-allergic mediator that inhibits the recruitment of mast cells into peripheral tissues. These observations are important for understanding mast cell pathophysiology and for the development of a therapeutic approach. SDF-1α has been shown to act as a chemoattractant for human MCps derived from cord blood mononuclear cells (MNCs) in vitro [22] , whereas another study reported that neutralization of SDF-1α or blockade of its receptor CXCR4 reduces airway allergic inflammation in vivo [29] . We report in this study that mast cells secrete both SDF-1α and PGD 2 , which positively and negatively modulate the infiltration of the mast cells themselves. Mast cell deficiency significantly reduced SDF-1α production in colon tissues; however, a wide range of cells, including epithelial and dendritic cells in addition to mast cells, may produce SDF-1α in colon tissue [30] , [31] . In addition, CXCR4 blockade reduced the infiltration of MCps in the H-PGDS −/− colon. These results suggest that SDF-1α is produced locally at the inflamed site, particularly by mast cells, and modulates further infiltration of MCps. Because we observed increased infiltration of mast cells but not of other types of cells into the H-PGDS −/− colon, we highlighted the effect of SDF-1α on MCps. However, SDF-1α is a powerful chemoattractant for various types of immune cells such as lymphocytes and monocytes [32] . Our data do not explain why hypersecreted SDF-1α accelerated the infiltration of only MCps. Interestingly, cofactors modulate the chemotactic effects of SDF-1α, depending on the cell type. Balabanian et al . [33] reported that IL-10 enhances the SDF-1α-induced chemotaxis of peritoneal B lymphocytes but not splenic B cells, whereas another study reported that histamine synergistically enhances the SDF-1α-induced migration of MCps but not mature mast cells or CD4 + T cells in vitro [34] . Therefore, there is a strong possibility that SDF-1α specifically recruits MCps cooperating with other mast cell-derived factors in allergic inflammation. Jeong et al . [35] demonstrated that mast cells are activated by the antigen-induced expression of hypoxia-inducible factor (HIF)-1α, a major transcription factor of SDF-1α (ref. 36 ). We have demonstrated that DP stimulation inhibits SDF-1α production in BMMCs. The DP receptor couples with Gs protein, and its activation increases the intracellular concentration of cAMP, which in turn inhibits the transcriptional activity of HIF-1α in human adenocarcinoma [37] . The PGD 2 -induced inhibition of SDF-1α production may result from inhibition of HIF-1α by DP signal activation. The activity of MMP-9 was also elevated, and its inhibition suppressed mast cell hyperplasia in the inflamed colon of H-PGDS −/− mice. MMP-9 cleaves pro-TNF-α and sheds membrane-associated SCF to activate the cytokines [20] , [21] . We did not detect a significant increase in TNF-α and SCF production in OVA-challenged colon tissues. However, at local inflammation sites in H-PGDS −/− mice, an increase in MMP-9 levels may promote the cleavage of TNF-α/SCF and thereby enhance the infiltration of MCps/mast cells. CXCR4 or MMP-9 inhibition exerts strong suppressive effects in H-PGDS −/− mice but not in WT mice. We previously reported that PGD 2 directly suppresses vascular hyperpermeability through the endothelial DP receptor in both lung inflammation and expanding tumour [38] , [39] . Another study demonstrated that the activation of DP receptors on dendritic cells increases levels of the anti-inflammatory cytokine, IL-10, in murine asthma [40] . In addition, activation of peroxisome proliferator-activated receptor-γ, which is the receptor of the dehydration product of PGD 2 , 15d-PGJ 2 , reduces the secretion of MMP-9 in an intestinal epithelial cell line [41] . Thus, PGD 2 may partially mediate other protective effects through a mast cell-independent pathway in allergic inflammation. Further investigation is needed to clarify these possibilities. We here demonstrated that endogenous PGD 2 signalling plays an anti-inflammatory role in allergic inflammation in vivo . In clinical settings, administration of nonsteroidal anti-inflammatory drugs, especially aspirin, is well known to enhance type I allergic reactions in the respiratory or GI tract [42] , [43] . Several studies have shown that aspirin enhances histamine and/or cys-LTs release from human leukocytes including mast cells [44] , [45] , [46] . However, aspirin also irreversibly inhibits the activity of COX-1, which plays a dominant role in PGD 2 production [47] . The inhibition of synthesis of the anti-inflammatory mediator PGD 2 by nonsteroidal anti-inflammatory drugs might be partially responsible for the enhancement. In conclusion, we have demonstrated that loss of PGD 2 exacerbates allergic inflammation and mast cell hyperplasia. Several diseases are accompanied by infiltration of mast cells, including allergy, inflammatory bowel disease and tumour [48] . Enhancement of PGD 2 signalling may be an effective treatment for these diseases. Mice All experiments were approved by The University of Tokyo’s Institutional Animal Care and Use Committee. Five- to eight-week-old female H-PGDS −/− (C57BL/6 and Balb/c) and littermates control mice or CXCR4 flox/flox mice (C57BL/6) were generated and bred as described previously [49] , [50] . Four-week-old female Kit W-sh/W-sh (C57BL/6) mice were generously provided by RIKEN BioResource Center. Food allergy model Five- to eight-week-old C57BL/6- and Balb/c mice were sensitized by intraperitoneal injection with 50 μg of OVA and 1 mg of aluminium potassium sulfate (Alum) in saline twice during a 2-week period. Following sensitization, OVA (50 mg: C57BL/6, 1 mg: Balb/c) was orally administered after 4 h of fasting, every other day. The allergic symptoms observed during a 45-min period after the challenges were scored as previously described [51] . The faeces score (0–2) was defined as follows: normal stool=0, soft stool=1 and loose or liquid stool=2. The systemic score (0–6) was defined as the sum of scores obtained from three criteria: scratching behaviour, loss of mobility and swelling. Scratching was graded based on the average number of scratching events during each 15-min interval (three intervals during a 45-min observation) as follows: 1–3 events=0, 4–5 events=1 and >6 events=2. Loss of mobility was graded according to immobility duration as follows: <10 min=0, >10 min=1, during the entire trial=2. Swelling (bristled fur, oedema around the nose and eyes, and laborious breathing) was graded as follows: none=0, swelling=2. For Balb/c mice, 1 mg of OVA was used to assess the allergic reaction because >10 mg of OVA induced a reaction that was too severe in H-PGDS −/− mice. The allergic reactions were assessed by diarrhoea occurrence (%) instead of faeces score, systemic score and hypothermia. Body temperature was measured using a rectal thermometer (Physitemp Instruments Inc., BAT-12) 30 min after OVA challenge. In the evaluation of Kit W-sh/W-sh mice, the systemic score excluding scratching was determined. In some experiments, the CXCR4 antagonist AMD3100 (300 μg per mouse in 100 μl saline) or the MMP-9 inhibitor MMP-9/MMP-2 inhibitor III (50 μg per mouse in 100 μl saline) was injected intraperitoneally before each OVA challenge. Morphological studies Dissected tissues were fixed in 4% paraformaldehyde for 24 h and embedded in paraffin. Sections (4 μm) were stained with CAE as previously described [52] . CAE-positive mast cells were counted in 20–25 randomly selected fields (× 400 magnification) per section. For immunohistochemistry, the colons were fixed for 2 h at 4 °C. Cryosections (4 μm) were incubated with PBS containing 0.05% Triton X-100 and 3% normal goat serum or bovine serum albumin for 15 min at room temperature. Antibodies such as rabbit-α-mouse H-PGDS (Cayman Chemicals, 1:500), rat-α-mouse c-kit (Merck Chemical, 1:125), hamster-α-mouse FcɛRI (1:125), rat-α-mouse CD4 (1:125), rat-α-mouse CD8 (Biolegend, 1:125) and rat-α-mouse CD11b (BD Biosciences, 1:125) were applied at 4 °C overnight. The secondary antibodies such as goat-α-rabbit Alexa 568, goat-α-rat Alexa 488 and goat-α-hamster Alexa 488 (Invitrogen, 1:500) were incubated at room temperature for 2 h. Images were captured using an Eclipse E800 fluorescence microscope (Nikon, Japan). H-PGDS- and/or c-kit-positive cells were counted in 10 randomly selected fields (× 400 magnification) per section from four independent experiments. Semiquantitative reverse transcription PCR Semiquantitative reverse transcription PCR was performed using SYBR Green Master Mix (Invitrogen) and specific primers ( Supplementary Table 1 ). Total RNA was isolated using Trizol reagent and reverse-transcribed to cDNA using ReverTra Ace (Toyobo). The real-time PCR was performed using an ABI7000 system (Applied Biosystems). Relative mRNA expression for each target was normalized to 18S ribosomal RNA values using the ΔΔCt method. MCp assessment The appearance ratio of MCps in colon tissue was determined by a limiting dilution assay. The dissected colons were chopped into 1-cm pieces and digested in 10 ml of RPMI containing 1 mg ml −1 collagenase IA (Sigma-Aldrich), 0.5 mg ml −1 dispase (Roche) and 0.2 mg ml −1 DNase I (Roche) at 37 °C for 75 min. The liberated cells were centrifuged over a two-step 44/67% Percoll gradient at 400 g for 20 min at room temperature. The MNC layer at the gradient interface was then harvested and the viable cells were counted. The MNCs (1 × 10 5 cells per ml) were used for four serial twofold dilutions with RPMI-1,640 containing 10% fetal bovine serum, 50 μM 2-mercaptoethanol and 10 ng ml −1 IL-3. Four different concentrations (1 × 10 5 , 5 × 10 4 , 2.5 × 10 4 and 1.25 × 10 4 cells per ml, 100 μl) of MNC dilutions were added to 24 wells of a standard 96-well flat-bottomed microtitre plate (Nunc). After a 10-day cultivation at 37 °C in 5% CO 2 , wells containing mast cell colonies were counted. The appearance ratio of MCps was calculated using L-Calc software Stemcell technologies. The ratio is expressed as the number of MCps per 10 6 MNCs. Measurement of PGD 2 The colons were homogenized using an amalgam mixer (Retsch, mm300) and mixed with 5 ml of ethanol containing 0.02% HCl at pH 2.0. After centrifugation at 500 g for 20 min, the supernatants were diluted with deionized water to 15% ethanol solutions, and PGD 2 -d 4 (100 ng ml −1 , internal standard) was then added. The solutions were applied to Sep-Pak Vac 3 cc cartridges (Waters) and the cartridges were washed with n -hexane. The analyte and internal standard were eluted from the cartridge with ethyl acetate. The eluate was dried and the residue was reconstituted in 10% (v/v) acetonitrile. The sample solution was then introduced into an LCMS-8030 system (Shimadzu) equipped with an electrospray (Turbospray) interface. The liquid chromatographic separation was conducted using a Kinetex C18 column (Phenomenex) using a mobile phase consisting of 0.02% (v/v) acetic acid (solvent A) and acetonitrile (solvent B). The following gradient was used at a flow rate of 400 μl min −1 : initial (2 min) at 95:5 (A:B), 10 min at 80:20, 18 min at 35:65 and 23 min at 10:90. The liquid chromatography-tandem mass spectrometry was operated in the negative ion mode. For analysis, the monitored transition for PGD 2 was m/z 351→271 and for PGD 2 -d4 it was m/z 355→319. PGD 2 was identified by elution time: 14.3 min. Isolation of BMMCs BM cells were collected from mouse femora and cultured in RPMI-1640 containing 10% fetal bovine serum, 50 μM 2-mercaptoethanol, 2 mM L -glutamine, 100 U ml −1 penicillin, 100 mg ml −1 streptomycin and 10 ng ml −1 IL-3 for up to 6 weeks at 37 °C in 5% CO 2 . To obtain CXCR4-deficient BMMCs, BMMCs isolated from CXCR4 flox/flox mice were incubated with a TAT Cre-recombinase (Merck Millipore, 2 μM) for 24 h at 37 °C in 5% CO 2 . Flow cytometric analysis showed that this procedure reduced the fraction of CXCR4-positive BMMCs to 10.2%. Chemotaxis assay The chemotactic response of BMMCs was examined using an 8-μm pore size insert chamber (BD Biosciences). Four-week-old BMMCs (1 × 10 6 cells per ml) in 400 μl of RPMI-1640 containing 25 mM HEPES and 0.1% bovine serum albumin were added to the upper insert chamber. The culture medium of 6-week-old BMMCs (diluted 1:50), SDF-1α (100 ng ml −1 ) or CCL-2 (10 ng ml −1 ) was added to the lower chamber. In some experiments, AMD3100 (10 μM) or RS504393 (10 μM) was added to both the upper and lower chambers 10 min before stimulation. After 5 h incubation, the migrated cells in the lower chamber were counted by means of flow cytometry. Adoptive transfer of BMMC to Kit W-sh/W-sh mice In the preliminary experiments, we administered WT or H-PGDS −/− BMMCs (6 weeks old, 1 × 10 7 ) to Kit W-sh/W-sh mice by tail-vein single injection as previously described [18] ( Supplementary Fig. 5a ). Six weeks later, the mice were sensitized with OVA in the same manner as described in the Food Allergy section. In the current study, after Kit W-sh/W-sh mice were sensitized with OVA, BMMCs (5 × 10 6 ) were injected into the tail vein of the Kit W-sh/W-sh mice 1 day before the first OVA challenge. BMMCs (1 × 10 6 ) were additionally injected every week after the first transplantation (multiple transfer; three times injections in total). Enzyme-linked immunosorbent assay All enzyme-linked immunosorbent assay procedures were performed according to the manufacturer’s instructions. For OVA-specific IgE (Biolegend) and mMCPT-1 (eBioscience) measurement, sera were collected from mice following the tenth challenge with either saline or OVA. For IL-3 (KOMAbiotech), IL-4 (Biolegend), SCF, SDF-1α (R&D Systems), IL-9, IL-13, TNF-α (eBioscience) and serotonin (Genway) measurements, whole-colon tissues obtained 24 h after the tenth OVA challenge were dissected and immediately frozen in liquid nitrogen. Frozen tissues were homogenized with amalgam mixer and suspended in PBS. After a 20-min centrifugation at 500 g , the supernatants were collected and used for enzyme-linked immunosorbent assay. For SDF-1α (R&D systems) and cys-LT (Enzo Life Sciences) measurements, the supernatants of BMMCs collected for the chemotaxis assay were used. Gelatin zymography Gelatin zymography was performed using a SDS–polyacrylamide gel containing 0.1% gelatin. The colon tissues were homogenized in lysis buffer (25 mM Tris-HCl, 0.1 M NaCl and 1% NP-40), and the extracts were electrophoresed on 8% polyacrylamide gels. After electrophoresis, the gels were incubated in 2.5% Triton X-100 for 30 min and incubated for 48 h at 37 °C in developing buffer (50 mM Tris-HCl, 0.2 M NaCl and 5 mM CaCl 2 ). The gel was then stained with 0.5% (w/v) Coomassie blue R-250 for 30 min. The band density of pro- (105 kDa) or active (act)-MMP-9 (95 and 88 kDa) was measured by ImageJ National Institutes of Health and shown as the ratio to WT. Electron microscopy Colon tissues were placed in a fixative containing 3% glutaraldehyde and 4% paraformaldehyde in 0.1 M phosphate buffer (pH 7.4) for 2 h at 4 °C. Following fixation, the tissues were rinsed in the same buffer and postfixed in 1% osmium tetroxide for 2 h at 4 °C. The tissues were then rinsed in distilled water, stained en bloc with 3% aqueous uranyl acetate overnight, dehydrated in a graded series of ethyl alcohol and embedded in Epon epoxy resin. Ultrathin sections were cut using a Reichert microtome and double stained with uranyl acetate and lead citrate before viewing with JEOL JEM 1200EX II and Hitachi H7000 electron microscopes. Data representation and statistical analysis All data are shown as the mean±s.e.m. Statistical significance of differences was determined by Student’s t -test for two-group comparisons by one-way analysis of variance with Tukey’s test or Dunnett’s test for multiple-group comparisons, and by the Mann–Whitney U -test for the faeces and systemic scores. How to cite this article: Nakamura, T. et al . PGD 2 deficiency exacerbates food antigen-induced mast cell hyperplasia. Nat. Commun. 6:7514 doi: 10.1038/ncomms8514 (2015).